Inconclusive evidence for rapid adaptive evolution 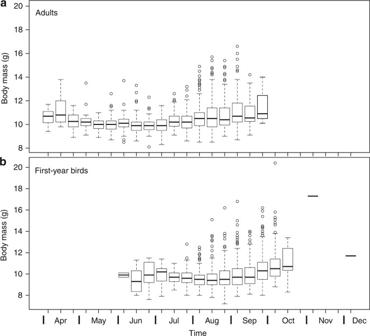Fig. 1 Boxplot depicting the seasonal variation in body mass ofaadult andbfirst-year reed warblers at Salreu, Estarreja and Portugal, during 1997–2014 (n= 1350 adults and 2535 first-years). This site is, as Malta, located in the southern part of the species’ breeding range (c. 550 km north of Malta, a difference that can be covered by migratory reed warblers in 1–3 days flight), but differs in having a very large population of local breeders. The greater body mass of migratory birds caught in April (spring/northward migration) and from August onwards (autumn/southward migration) is obvious despite the fact that (i) only first captures are included here (recaptures show large increases in body mass during the migratory periods); and that (ii) local birds are particularly small (have a low body mass) and abundant, and are breeding almost until the end of August (a period when they are still lean). Indeed, pre-migratory fattening of local birds and the arrival of migrants from the north has been widely described to occur in August at these latitudes3. Consequently, between 1 May and 31 August (i.e. during Sætre et al.’s1sampling period), the body mass of both adults and juveniles caught in Portugal varies highly significantly with date (Adults: Mass = 10.29311 − 0.01603Date + 0.00019Date2,F2;1193= 70.08,P= 2.2e−16, df = 1193,R2= 0.1051; First-years: Mass = 11.77166 − 0.04875Date + 0.00026Date2,F2;1375= 8.162,P< 0.001, df = 1375,R2= 0.01173) 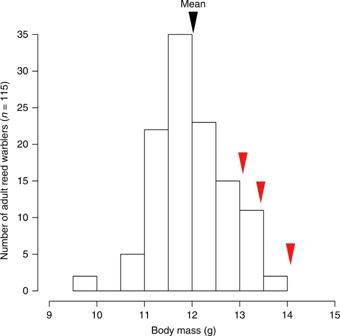Fig. 2 Histogram of body mass of all 115 adult reed warblers in Krankesjön, southern Sweden, during May–August 2013–2016, showing the average for this population (black triangle), and the averages of body mass for the first 3 years of Sætre et al.1study (red triangles). Although Swedish reed warblers are larger than south-European individuals (e.g. compare with data in Fig.1), the average body mass of the birds caught by Sætre et al.1in Malta during the first 3 years of their study largely exceeds the one for Scandinavian birds, and data from the first year of their study even exceeds the total variation depicted in this histogram. This strongly suggests that a high proportion of migratory birds, which have a large amount of fat reserves, were included in their data set Sampling The capture and ringing of birds were conducted under the licenses required by the corresponding national authorities, following standard protocols and releasing the birds unharmed on site. In particular, reed warblers were caught with mist-nets, marked with an aluminium ring issued by the ringing centres of Portugal (CEMPA, ICNF; ringing permits 68/97, 68/98, 45/99, 55/2000, 62/2001, 69/2002, 67/2003, 71/2004, 73/2005, 75/2006, 82/2007, 88/2008, 86/2009, 92/2010, 99/2011, 112/2012, 118/2013) or Sweden (Naturhistoriska riksmuseet, Stockholm; ringing permit 683). Among other measurements, birds were weighed using a digital or a Pesola spring balance to the nearest 0.1 g. In Krankesjön, Skåne, Sweden, 95% of the birds were caught using a constant-effort method, that is, using the same net positions, location and time of day, and during 12 sessions each year evenly distributed from the beginning of May to the end of August; which coincides with Sætre et al.’s [1] sampling period. Only the first capture of each bird was used to avoid pseudo-replication. The effect of date of capture (1 = 1 May) on body mass was evaluated using a linear regression model in which the quadratic term was included as it lowered the AIC (by more than 10). Data availability The data are available in Supplementary Data 1 .